UnencapsulatedStreptococcus pneumoniaefrom conjunctivitis encode variant traits and belong to a distinct phylogenetic cluster Streptococcus pneumoniae , an inhabitant of the upper respiratory mucosa, causes respiratory and invasive infections as well as conjunctivitis. Strains that lack the capsule, a main virulence factor and the target of current vaccines, are often isolated from conjunctivitis cases. Here we perform a comparative genomic analysis of 271 strains of conjunctivitis-causing S. pneumoniae from 72 postal codes in the United States. We find that the vast majority of conjunctivitis strains are members of a distinct cluster of closely related unencapsulated strains. These strains possess divergent forms of pneumococcal virulence factors (such as CbpA and neuraminidases) that are not shared with other unencapsulated nasopharyngeal S. pneumoniae . They also possess putative adhesins that have not been described in encapsulated pneumococci. These findings suggest that the unencapsulated strains capable of causing conjunctivitis utilize a pathogenesis strategy substantially different from that described for S. pneumoniae at other infection sites. S treptococcus pneumoniae is a leading cause of invasive infections including pneumonia, meningitis and sepsis, as well as noninvasive infections including pharyngitis and otitis media. The polysaccharide capsule, a key virulence factor, is the target of current vaccines [1] , [2] , [3] . Vaccination has substantially reduced morbidity and mortality [3] but has had limited impact on conjunctivitis, infection of the mucous membrane covering the eye and lining the eyelids [4] . We recently collected 271 S. pneumoniae isolates during the course of clinical trials for the treatment of bacterial conjunctivitis [5] , [6] , [7] and found that over 90% were unencapsulated [8] , and hence unaffected by current vaccine design. Unencapsulated S. pneumoniae strains have caused large conjunctivitis outbreaks in schools and colleges [9] , [10] , [11] , [12] , [13] , military training facilities in the United States [14] and at other locations worldwide [15] . Recent outbreaks have involved one multilocus sequence type (MLST) in particular, ST448 (ref. 13 ). However, a previous study of epidemiologically unrelated conjunctivitis cases found that most cases were caused by encapsulated strains [4] . That study examined isolates before the widespread use of the PCV7 vaccine introduced in 2000 (ref. 4 ). With a view towards assessing the impact of the vaccine and improved vaccine design, and to better understand the diversity of strains and genetic basis for S. pneumoniae pathogenesis in conjunctivitis, here we describe the results of an extensive comparative analysis of S. pneumoniae currently associated with conjunctivitis. Epidemiology of conjunctivitis To determine the diversity of S. pneumoniae causing conjunctivitis, 271 strains [5] , [6] , [7] , [8] were characterized by MLST [16] ( Fig. 1 , Supplementary Data 1 ). Sequence type ST448 (refs 17 , 18 ) was found to cause the majority of infections (67.2%). The next most common types caused substantially fewer: ST344 (8.9%), ST1186 (4.8%) and ST2315 (4.4%). Together, 10 different sequence types of unencapsulated S. pneumoniae accounted for 90.8% of conjunctivitis cases. A diverse set of strains of S. pneumoniae from other types of infections, for which closed genomes are available in Genbank, were included for comparison ( Supplementary Data 2 ). A distinct, deeply rooted cluster of S. pneumoniae was formed that included 11 unencapsulated MLST types encompassing 89.3% of conjunctivitis isolates ( Fig. 2 ). Only one sequence type that is encapsulated, ST199, caused more than two cases. This shows that conjunctivitis in the United States is mainly caused by a closely related group of unencapsulated S. pneumoniae sequence types, although other strains can cause conjunctivitis, most likely as an extension of upper respiratory infection. 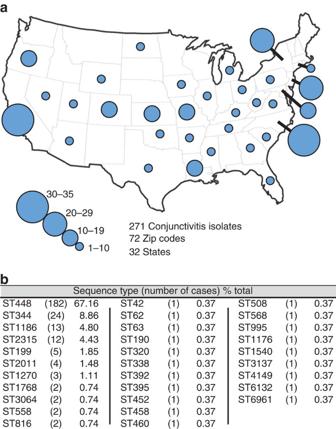Figure 1: Location and MLST profile of conjunctivitis isolates. Two hundred seventy-one isolates ofS. pneumoniaefrom diagnosed cases of conjunctivitis. (a) Number and geographic location of isolates. (b) Frequency of MLST types among conjunctivitis isolates. Figure 1: Location and MLST profile of conjunctivitis isolates. Two hundred seventy-one isolates of S. pneumoniae from diagnosed cases of conjunctivitis. ( a ) Number and geographic location of isolates. ( b ) Frequency of MLST types among conjunctivitis isolates. 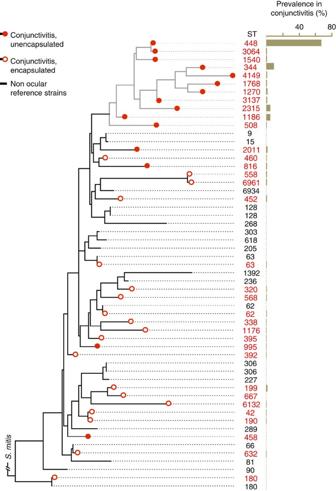Figure 2: MLST-based phylogenetic relationships among conjunctivitis strains. SNP-based tree based on a concatenation of MLST loci, with prevalence in conjunctivitis for each ST. Full size image Figure 2: MLST-based phylogenetic relationships among conjunctivitis strains. SNP-based tree based on a concatenation of MLST loci, with prevalence in conjunctivitis for each ST. Full size image Traits of the unencapsulated conjunctivitis cluster To determine whether strains from conjunctivitis that occur within the distinct branch of S. pneumoniae possess novel gene content, a total of 21 genomes of representatives of the major conjunctivitis-associated sequence types were sequenced ( Supplementary Data 3 ). Diversity was maximized by selecting varying dates of isolation and sites of origin. In addition, genomes of select encapsulated conjunctivitis strains were also sequenced, including ST199 (which caused five cases) and strains of sequence types ST632, ST667 and ST180. Genes encoding a total of 4,433 protein orthogroups were identified by OrthoMCL, 1,160 of which were present in single copy in all genomes. These core orthogroup genes were used to generate a single-nucleotide polymorphism (SNP)-based phylogenetic tree ( Fig. 3 ). As for MLST, the SNP-based core genome tree showed that strains isolated from epidemic conjunctivitis belong to a distinct, deeply resolved group that includes ST448, ST1186, ST344, ST1270 and ST2315. Lineages within this group were termed the epidemic conjunctivitis cluster (ECC), since their genomes are highly related and these STs (ST448, ST344 and ST1186) are associated with epidemic conjunctivitis outbreaks [9] , [10] , [14] , [17] , [18] . Croucher et al. [19] recently noted that one group of unencapsulated strains (denoted Sequence Cluster 12 (SC12)) was the most divergent cluster from the main population in their study. SC12 includes STs ST448 and ST344 associated with conjunctivitis. The phylogeny determined here was unchanged after filtering recombinogenic regions of DNA using BRAT NextGen [20] , showing that recombination was not the main driver for this population structure. Encapsulated strains that are rarer causes of conjunctivitis (ST632, ST667, ST180 and ST199) are interspersed among strains that cause infection at other sites. The extent of divergence of shared genes within ECC genomes from those of other sites of infection was quantified [21] ( Supplementary Fig. 1 ). ECC genomes compared with each other exhibit an average nucleotide identity (ANI) value of 99.0% ±0.4, highlighting the very close relationship among ECC lineages. ECC strains are significantly more distantly related to those from other sites of infection (97.9% ±0.11 ANI, P <0.001, Student’s t -test). 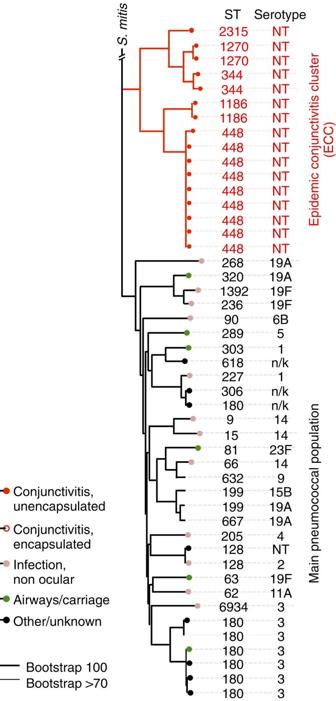Figure 3: ECC strains belong to a well-resolved group of the speciesS. pneumoniae. A PhyML SNP-based tree based on the concatenated alignments of 1,160 single-copy core genes (for strain identities, seeSupplementary Data 2). Bootstrapping was performed with 1,000 iterations. Figure 3: ECC strains belong to a well-resolved group of the species S. pneumoniae . A PhyML SNP-based tree based on the concatenated alignments of 1,160 single-copy core genes (for strain identities, see Supplementary Data 2 ). Bootstrapping was performed with 1,000 iterations. Full size image ECC strains possess a distinct gene repertoire Clustering of genomes based on similarities in gene content also places ECC strains into a well-resolved group, independently recapitulating phylogenic structure ( Supplementary Fig. 2 ) and supporting the hypothesis that the peculiar ocular tropism of ECC strains stems at least in part from novel gene content. As in the SNP-based phylogeny, strains that are rarer causes of conjunctivitis are interspersed among non-ocular S. pneumoniae . To identify genes that distinguish the ECC from other strains, because horizontal gene flow can complicate the analysis, we arbitrarily set gene presence in 80% or greater of ECC genomes, and <20% of the non-ECC comparator strains (or vice versa ) as the cutoff. We found 230 genes that fulfil this enrichment criteria ( Supplementary Data 4 ). Of these, 103 genes are in all ECC genomes and absent from all comparators. Conversely, 70 genes are missing from ECC that are present in 80–100% of non-ocular S. pneumoniae comparator genomes ( Supplementary Data 5 ). Of those, 29 were found in all non-ocular genomes and no ECC strains. In patterns of gene presence and absence, encapsulated conjunctivitis strains were found to be most closely associated with those from other types of infection. The comparatively large proportion of conjunctivitis caused by ST448 suggests that its genome may be especially refined to cause this disease (or alternatively, that among ECC lineages, ST448 is more widely distributed and abundant in nature). Seventeen orthogroups are unique to ST448 ( Supplementary Data 6 ), including a hypothetical mobile element with closest relative in S. mitis. No genes are specifically missing from ST448 that are in all other ECC genomes. Evidence for large-scale surface remodelling In place of a capsule operon, all ECC strains we investigated possess the atypical locus that includes aliC (X231_0947) and aliD (X231_0948) but not the often-associated pspK gene [22] , [23] . However, in the absence of a capsule, a large number of novel surface features were found. Exclusive to ECC are two different Antigen I/II family adhesins (X231_1085 and X231_1187; Supplementary Data 4 ) that appear to originate from S. macedonicus and S. mitis , respectively ( Fig. 4a ). Owing to the presence of multiple SspB domains within these proteins, we termed them SspBC1 (X231_1085) and SspBC2 (X231_1187). SspB domain-containing proteins have been shown to bind the human scavenger protein gp-340, which contributes to bacterial aggregation [24] . To test for this functionality, a representative ECC strain (ST448), and a non-ECC-encapsulated conjunctivitis strain that lacks SspBC1 and SspBC2 (ST199), were incubated with graded concentrations of gp-340. As shown in Fig. 4b , the ST448 strain exhibited gp-340 concentration-dependent aggregations. We also identified a unique gene inferred to encode a surface protein (X231_1186) termed here PspO. This surface protein gene is directly adjacent to that encoding SspBC2, suggesting a potential virulence island. PspO includes a C-terminal glucan-binding domain and a surface exclusion domain. 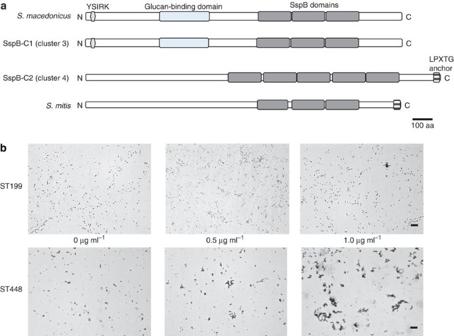Figure 4: Homologues of agglutinin receptors in ECC. (a) SspBc1 and SspBc2 agglutinins exhibit identity to glucan-binding and SspB domains in orthologues fromS. macedonicusorS. mitis. (b) Aggregation of ST448 (ECC_3540) and ST199 (SC_3526) isolates after addition of 0.5 and 1.0 μg ml−1of gp-340 visualized with Gram staining. Scale bar represents 20 μm. Figure 4: Homologues of agglutinin receptors in ECC. ( a ) SspBc1 and SspBc2 agglutinins exhibit identity to glucan-binding and SspB domains in orthologues from S. macedonicus or S. mitis . ( b ) Aggregation of ST448 (ECC_3540) and ST199 (SC_3526) isolates after addition of 0.5 and 1.0 μg ml −1 of gp-340 visualized with Gram staining. Scale bar represents 20 μm. Full size image Another gene predicted to affect the host/pathogen interface, that occurs exclusively in ECC strains, encodes a new divergent putative zinc metalloprotease (X231_0594), ZmpC2 ( Supplementary Fig. 3A ). The closest orthologue is in S. pseudopneumoniae IS7493, and it shares 31% amino-acid sequence identity with the known ZmpC of S. pneumoniae , mainly in the Peptidase_M26_C domain ( Supplementary Fig. 3A ). Recently, a different, structurally related, atypical zinc metalloprotease C ( zmpC, now termed ZmpC1) was identified in a S. pneumoniae conjunctivitis isolate, and was shown to cleave mucins from corneal epithelial cells [25] , [26] . ZmpC1 (X231_0222) also occurs in 100% of ECC and 0% of comparators. Additional surface-related functions of potential relevance to conjunctivitis include a putative sialidase (X231_0534), now termed NanO1. It shares 88% amino-acid sequence identity with sialidase A (neuraminidase A) of S. pseudopneumoniae . The typical NanA of S. pneumoniae , which is carried by all non-ocular reference strains, has been displaced by NanO1 in ECC ( Supplementary Fig. 3B ). Closer examination of the sequence surrounding nanO1 identifies a second gene, also annotated as encoding a sialidase (referred to as NanO2, X231_0533), suggesting that NanO1 and NanO2 from S. pseudopneumoniae recombinationally displaced wild-type NanA ( Supplementary Fig. 3C ). In addition, the neuraminidase allele NanC, found in ~51% of S. pneumoniae isolates from non-ocular sites [27] , was not found within any ECC genome. Choline-binding proteins (Cbps) are important virulence factors that contribute to S. pneumoniae adhesion and transcytosis [28] . All ECC genomes encode a novel, divergent Cbp (BM49_0273), CbpI1, that is most closely related to a variant in S. pseudopneumoniae . All ECC strains also encode a second Cbp variant (X231_0220, CbpI2) that is rare outside this cluster, occurring in three non-ocular comparator strains (AP200, G54 and TIGR4) [28] . CbpI1 and CbpI2 share a structurally related cysteine-rich secretory domain and a C-terminal choline-binding domain, and 48.3% overall amino-acid sequence identity. Interestingly, CbpI2 and ZmpC1 are adjacent to one another within the ECC genomes. S. pneumoniae genes with known roles in colonization and virulence include cbpA, nanB, bgaA, strH, ply, hyl, plpA (aliA), psaABC, prtA, choP, pdgA, adr, spxB, amiA-amiF, msrA/B2 and the two Pilus Islets [29] , [30] , [31] . Choline-binding protein A (CbpA), a main adhesin in respiratory infections and otherwise highly conserved in non-ocular strains [31] , [32] , is substantially divergent in all ECC genomes. Two polymorphic forms of CbpA were found, CbpAC1 in ST448 and ST1186 genomes, and CbpAC2 in ST344, ST1270 and ST2315 ( Fig. 5 ). Portions of CbpAC1 and CbpAC2 show little resemblance to CbpA, instead being closely related to the beta antigen of S. agalactiae [33] . The absence of CbpA from ECC strains was verified with western blot analysis using three different CbpA-specific monoclonal antibodies [34] , indicating that the variant CbpA possesses a substantially different structure in the otherwise conserved key epitopes probed ( Supplementary Fig. 4 ). The region of canonical CbpA that mediates binding to the eukaryotic polymeric Ig receptor [35] has been replaced by S. agalactiae domains that bind the Fc portion of IgA directly [33] , [36] . The different variations in the divergence of CbpAC1 and CbpAC2 from CbpA suggest that variations of the hybrid CbpA locus evolved independently. Interestingly, in ECC the two-component system that regulates CbpA expression [37] also exhibits greater nucleotide sequence identity to its counterpart in S. agalacticae ( Supplementary Fig. 4D ). Differences in nucleotide sequence on either side of the two variant CbpAC loci support separate evolution of these determinants within ECC strains. 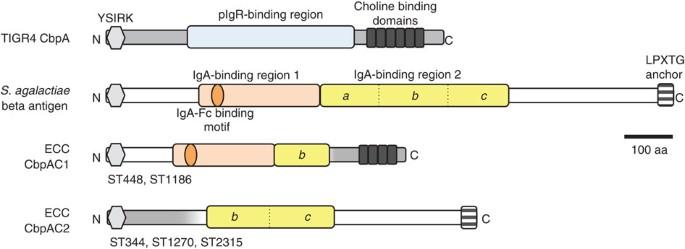Figure 5: ECC genomes encode an atypical CbpA. Canonical CbpA of TIGR4 compared with those in ECC genomes, and the inferred donor,S. agalactiaeC beta antigen. Sequence most likely deriving fromS. pneumoniae(grey) andS. agalactiae(white). Domains relevant to polymeric Ig receptor (pIgR) or IgA-binding are highlighted. The IgA-binding domain ofS. agalactiaebeta antigen is duplicated, and domain 2 has been divided into portions (a, b, c) for purposes of illustrating the likely origins of fragments that share amino-acid sequence identity in ECC variants. Figure 5: ECC genomes encode an atypical CbpA. Canonical CbpA of TIGR4 compared with those in ECC genomes, and the inferred donor, S. agalactiae C beta antigen. Sequence most likely deriving from S. pneumoniae (grey) and S. agalactiae (white). Domains relevant to polymeric Ig receptor (pIgR) or IgA-binding are highlighted. The IgA-binding domain of S. agalactiae beta antigen is duplicated, and domain 2 has been divided into portions (a, b, c) for purposes of illustrating the likely origins of fragments that share amino-acid sequence identity in ECC variants. Full size image Two pilus islets have been described that contribute to S. pneumoniae epithelial cell adhesion [29] , [30] . Neither pilus islet occurred in any ECC strain. Exoglycosidase BgaA is absent from all ECC isolates, as is a three-gene phosphotransferase system (PTS) (SP_0645 to SP_647) that occurs immediately adjacent to bgaA in TIGR4, displaced by ~1 kb of sequence with high identity (>91%) to sequences in S. mitis and S. pseudopneumoniae . Otherwise, all other virulence-associated genes, including nanB, strH, ply, hyl, plpA (aliA), psaABC, prtA, choP, pdgA, adr, spxB, amiA-amiF and msrA/B2 are present in all ECC strains, and are highly conserved (99.6% ±0.3 inferred amino-acid sequence identity to TIGR4). Metabolic differences All ECC strains encode a putative phosphoenolpyruvate-dihydroxyacetone phosphotransferase system (X231_1297 to X231_1300, Supplementary Data 4 ). Uniformly absent from ECC strains are operons for arginine metabolism (SP_2148 to SP_2151), and a fucose-binding, uptake and catabolic pathway (SP_2158 to SP_2170) ( Supplementary Data 5 ). This block of metabolic functions has been displaced in ECC genomes with a 12.7-kb sequence that encodes, among other things, ZmpC2. Some ECC (ST448, ST344 and ST1270) lack the pia operon-mediating iron uptake, which in other strains has been linked to virulence in mouse models of pulmonary and systemic infection [38] . Five other genes with putative annotations as amino-acid transporters (SP_0111, SP_0112 and SP_0709 to SP_0711) are present in 100% of comparators, but are uniformly absent in ECC, suggesting a substantially altered nutrient profile in the conjunctival mucosa ( Supplementary Data 5 ). Recombination and horizontal gene transfer The occurrence of multigene blocks of difference suggests that movement of pathogenicity islands or other mobile elements were involved in the evolution of ECC. Of the 230 orthogroups enriched in ECC, 180 genes occur in 15 clusters ( Table 1 ). The average G+C content (36.8% ±3.8) is lower than the rest of the genome (39.7%, P <0.01, Student’s t -test), which is common for mobile elements [39] . Two clusters exclusive to ECC, an 18-kb predicted phage (cluster 9) and 13-kb encoding core genes (VirD/VirB/TrsE) of a Type IV secretion system (cluster 11), are adjacent. Interestingly, the cluster 9/cluster 11 element occurs at different locations within ECC STs, suggesting either independent acquisition or internal movement. That it is mobile and presumably could be lost if not for selection, yet is retained, suggests that it may have a role in mediating the peculiar ocular tropism of ECC. Table 1 Gene clusters enriched in ECC genomes. Full size table The majority (75%) of ECC carry resistance elements ( Supplementary Fig. 5 ) consistent with antibiotic susceptibility [40] . Macrolide resistance is the most common, and is conferred by the Macrolide Efflux Genetic Assembly cassette in ST448 and ST1186, and by a Tn916-like integrative conjugative element in ST344 and ST1270 ( Supplementary Fig. 6 ). ST2315 was the only ECC isolate resistant to phenicols, which was conferred by an Spn11930-like integrative conjugative element element. Comparison with strains identified in asymptomatic carriage Asymptomatic nasopharyngeal carriage generally precedes disease. To determine whether ECC strains were represented in large data sets from asymptomatic carriage, we looked for their occurrence in two recently reported studies [19] , [41] . This expanded analysis substantiates the deeply rooted and well-clustered grouping of the ECC strains but, importantly, shows that ECC STs are distributed among additional closely related, unencapsulated strains isolated from the nasopharynges that have not yet been associated with conjunctivitis ( Fig. 6 ). It was thus of interest to compare the traits of ECC strains isolated from conjunctivitis to those isolated from the nasopharynx by investigating the presence or absence of a selection of newly identified ECC genes with a putative contribution to conjunctivitis pathogenesis. From the asymptomatic carriage data sets, we selected genome sequences of 96 strains that were of sequence types closely related to those that constituted the ECC group, and also diverse strains spread across the phylogenetic tree representing the most prevalent STs associated with nasopharyngeal carriage regardless of their encapsulation status ( Fig. 6 , Supplementary Fig. 7 and Supplementary Data 7 ). All genes found to be enriched in ECC strains isolated from conjunctivitis were also found to be present within nasopharyngeal isolates of ST448, ST2315 and ST344 genomes, indicating that these strains are highly similar to those isolated from conjunctivitis, and supporting an infection model where asymptomatic carriage in the nasopharynx precedes ocular infection. Of the cumulative 3,701 nasopharyngeal isolates represented in the two nasopharyngeal surveys, no representatives of ST1186 or ST1270 were observed, in contrast to their occurrence at rates of 13/271 (4.8%) and 3/271 (1.1%), respectively, in conjunctivitis cases, indicating their rarity among the circulating population despite their enrichment in cases of conjunctivitis. 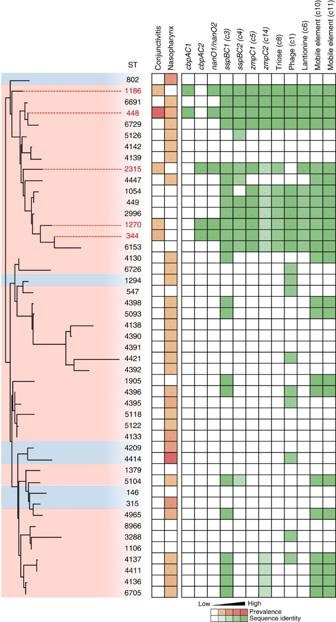Figure 6: Presence of ECC genes in genomes of nasopharyngeal isolates. All STs representative of unencapsulated strains (pink highlight), and the most prevalent encapsulated strains (blue highlight), from two recent large-scale surveys of asymptomatic nasopharyngeal carriage19,41, compared with ECC members associated with conjunctivitis (red text and line extension), shown in a PhyML SNP-based tree based on the concatenated alignments of MLST alleles. Bootstrapping was performed with 1,000 iterations. Prevalence in conjunctivitis (this study) and nasopharyngeal carriage41is shown. Percent presence and sequence identity of gene (gene, cluster number) or cluster (predicted function, cluster number) is denoted with green boxes. Figure 6: Presence of ECC genes in genomes of nasopharyngeal isolates. All STs representative of unencapsulated strains (pink highlight), and the most prevalent encapsulated strains (blue highlight), from two recent large-scale surveys of asymptomatic nasopharyngeal carriage [19] , [41] , compared with ECC members associated with conjunctivitis (red text and line extension), shown in a PhyML SNP-based tree based on the concatenated alignments of MLST alleles. Bootstrapping was performed with 1,000 iterations. Prevalence in conjunctivitis (this study) and nasopharyngeal carriage [41] is shown. Percent presence and sequence identity of gene ( gene , cluster number) or cluster (predicted function, cluster number) is denoted with green boxes. Full size image Genes we identified as enriched in ECC strains isolated from conjunctivitis, cbpAC1 , cbpAC2 and nanO1/nanO2 , were only found to occur among asymptomatic carriage strains of the same sequence types. Other genes that we found to be enriched in ECC (sspBC1, sspBC2, zmpC1 and zmpC2 ) also occurred in unencapsulated lineages that have not yet been observed in conjunctivitis, and the majority of these lineages are closely related phylogenetically to ECC strains ( Fig. 6 ). Interestingly, some sequence types phylogenetically closely related to ECC strains (ST5126, ST4142 and ST4139) were found to lack all ECC genes that were investigated. As these STs were not identified among conjunctivitis strains, their ability to cause this disease remains unknown. With a view towards understanding strain diversity and the molecular basis for virulence of S. pneumoniae in conjunctivitis, and to improving vaccine design to cover this disease, we characterized recent isolates from across the United States. We found that nearly 90% of conjunctivitis cases were caused by five related STs (ST448, ST344, ST1186, ST1270 and ST2315) that occur within a distinct cluster of the S. pneumoniae species (see Fig. 6 and Supplementary Fig. 7 ), a population structure supported by two recent reports [19] , [41] . This divergence is characterized by novel gene content constituting ~10% of the genome. Although ECC strains possess a large amount of novel genes, shared genes exhibit an ANI of 97.9% ±0.11 ANI with strains from other types of infection, and therefore ECC strains do not constitute a new species (ANI<95%) by this definition [19] , [21] , [42] . We found that genes cbpAC1 , cbpAC2 , nanO1 and nanO2 were only carried by STs that are associated with conjunctivitis (see Figs 6 and 7 ). Other genes enriched in ECC, including the sspBC agglutinins, zmpC1 , zmpC2 and the triose metabolic cassette, were found to be shared among a few closely related unencapsulated STs (ST6153, ST6691, ST6729, ST2996, ST1054 and ST449) that have not been identified in cases of conjunctivitis, which may stem from the paucity of studies that have identified MLST types of S. pneumoniae causing conjunctivitis. These additional genes are largely absent in encapsulated and more distantly related unencapsulated genomes unrelated to conjunctivitis however (see Figs 6 and 7 ). These findings suggest that some of the genes enriched in ECC are fundamental to the formation of the larger unencapsulated lineage to which ECC members belong (see Fig. 6 and Supplementary Fig. 7 ). 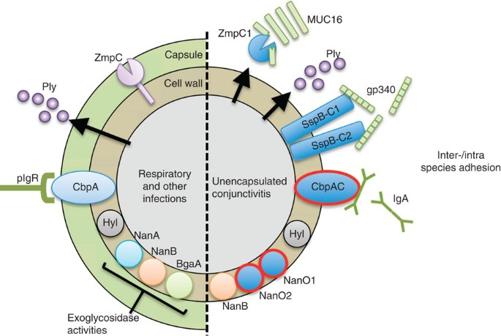Figure 7: Virulence factor differences between invasive and ECC strains. New traits found within ECC and closely related genomes are shown in solid blue, with those unique to STs associated with conjunctivitis highlighted with red outline. CbpAC1 and CbpAC2 are shown as CbpAC, since ECC strains express one or the other, but not both. Predicted ligands for SspBC1, SspBC2 and CbpAC are shown. Host-derived molecules are illustrated in green. Arrows indicate secreted products. Figure 7: Virulence factor differences between invasive and ECC strains. New traits found within ECC and closely related genomes are shown in solid blue, with those unique to STs associated with conjunctivitis highlighted with red outline. CbpAC1 and CbpAC2 are shown as CbpAC, since ECC strains express one or the other, but not both. Predicted ligands for SspBC1, SspBC2 and CbpAC are shown. Host-derived molecules are illustrated in green. Arrows indicate secreted products. Full size image Typifying the conjunctivitis-associated strains is a lack of capsule, rendering them unaffected by current polyvalent pneumococcal capsule vaccines. As would be predicted for a lineage that professionally lacks the polyanionic capsule through which surface proteins must fold and extend, these strains have substantially different surface features, including those known to contribute to virulence ( Fig. 7 ). Novel features, specific to ECC STs include substantially altered forms of CbpA, CbpAC1 and CbpAC2. Interestingly, these no longer possess the key domain that mediates binding to host polymeric Ig receptor, which S. pneumoniae use to facilitate transcytosis from nasopharyngeal epithelia into the blood stream [35] . Instead, both CbpAC1 and CbpAC2 appear to have independently swapped that domain for one that mediates direct binding to secretory IgA [33] , [36] , [43] . The implication is that ECC strains bind secretory IgA in a subtly, but importantly, different way, possibly coating themselves with IgA, in a manner analogous to that mediated by protein A of S. aureus [44] . Alternatively, these CbpA variants may act as adhesins for attachment to surfaces coated with antibodies, as suggested for immunoglobulin receptors in S. pyogenes [45] . That this change appears to have occurred twice, and that only variants of CbpA occur in unencapsulated STs associated with conjunctivitis, suggests that it is important for the ocular tropism. In addition to the variant CbpA, all ECC genomes also encode two novel, divergent choline-binding protein CbpI’s, here termed CbpI1 and CbpI2. No function has yet been ascribed to CbpI, CbpI1 or CbpI2. Other factors unique to STs associated with conjunctivitis that could affect the host/microbe interface include the displacement of NanA with two variant sialidases, NanO1 and NanO2. This recombination event is seen only in ECC members and is absent even in the closest non-ECC relatives. Since sialic acid residues exhibit variation among host cell types, it has been suggested that they are mediators of tissue tropism [46] . This is of potential relevance to conjunctivitis, since proteins found at the ocular surface are decorated by covalently bound sialic acids [47] , which have been shown to mediate ocular surface binding of Pseudomonas aeruginosa and Escherichia coli [48] , [49] . A recurring motif was the replacement of surface features optimized for function in the presence of a capsule, with surface features derived from unencapsulated oral streptococci (for example, S. mitis ). Others have noted that S. mitis appears to be a reservoir of genetic diversity [50] . Additional novel surface features of ECC and closely related unencapsulated strains likely involved in colonization, and likely originating in oral streptococci, include two Antigen I/II (AgI/II) family of adhesins/agglutinins encoded in separate genomic islands, SspBC1 and SspBC2. Notably, sspBC2 is restricted to ECC and closely related strains potentially implicating its involvement in the unusual ocular surface tropism, whereas sspBC1 is also found within more distantly unencapsulated genomes, implicating its possible involvement in colonization of the nasopharynx and adnexa (see Fig. 6 ). The AgI/II family of adhesins is central to colonization and biofilm formation by commensal and pathogenic species of Streptococcus [24] , [51] . A previous review noted their ubiquitous presence among streptococci except for S. pneumoniae [51] . The observation here that these genes occur in unencapsulated strains of S. pneumoniae suggests either incompatibility or functional redundancy with the pneumococcal capsule. In terms of colonization (nasopharyngeal and/or ocular) and conjunctivitis pathogenesis, SspB domains of AgI/II proteins mediate binding to human scavenger protein gp-340 (ref. 24 ), which occurs in tears and on the ocular surface [52] . All STs associated with conjunctivitis encoded a novel phage element (cluster 9/cluster 11). This element was also seen in closely related unencapsulated nasopharyngeal strains, whereas it was rarely found in more distantly related unencapsulated strains. Interestingly, this element is located at different sites in the genomes of the conjunctivitis-associated sequence types but is always consistent within an ST. This suggests that it was lacking from a common ancestor and has been acquired independently, or that it is internally mobile. There are no obvious adhesins or virulence traits encoded within this element; however, it may contribute to biofilm formation as described for other phage elements in S. pneumoniae [53] . Its presence within numerous nasopharyngeal STs suggests that it may play a basic function in colonization for unencapsulated varieties of S. pneumoniae . A unique metabolic feature profile was found among ECC and closely related strains, suggesting that their colonization ability is likely nutritionally distinct from that of strains associated with invasive infection. A phosphoenolpyruvate-dihydroxyacetone PTS gene cluster occurring in ECC and closely related nasopharyngeal strains and only one distantly related strain from otitis media (Hungary19A-6, cluster 8), also found in S. mitis and S. pseudopneumoniae , suggests that the ability to metabolize Dha is important for mucosal surface colonization. DhaP was detected among the phosphorylated intermediate metabolites present on the ocular sclera and corneal tissues [54] . In addition to the gain of putative metabolic capabilities described above, all ST genomes associated with conjunctivitis lacked the ability to metabolize fucose, a sugar that decorates ocular glycans present in the glycocalyx of corneal epithelial cells [49] . Fucosylated glycans coating mucins are known to promote bacterial colonization in the gut, serving as both adherence targets, as well as a carbon source [55] , [56] . Specifically at the ocular surface, fucose residues have been implicated in the attachment of P. aeruginosa and E. coli to ocular epithelial cells [49] . Moreover, application of exogenous fucose was shown to suppress inflammation in rabbit corneal and explanted human cornea models of wound-healing [57] . Nasopharyngeal STs closely related to ECC members (ST6691, ST6729, ST1054, ST449, ST2996 and ST6153) were also found to lack the elements to metabolize fucose. These findings suggest that the inability to metabolize fucose is irrelevant for colonizing the nasopharynx but may confer an advantage at the ocular surface, potentially by promoting an anti-inflammatory environment and/or by preserving an important bacterial ligand. While asymptomatic carriage in the nasopharyngeal cavity is likely to be a precursor to infection, ST448 (refs 9 , 12 , 13 , 15 , 18 ) and related STs commonly isolated conjunctivitis were not highly prevalent in recent large-scale surveys of asymptomatic S. pneumoniae carriage in the nasopharynx [19] , [41] . Whereas ST448 was found to be by far the leading cause of conjunctivitis in this study as well as in others [15] , [18] , it represented only 1.43% of 3,084 isolates found to be asymptomatically carried by Chewapreecha et al. [41] , and 1.14% of nasopharyngeal isolates examined by Croucher et al. [19] Indeed, there are four other unencapsulated STs found at similar or higher prevalence within the nasopharynges (ST4133, ST4395, ST4965 and ST4136 ranging from 1.43 to 2.92%), the most prevalent of which, ST4133, has not been reported as a cause of conjunctivitis, is not closely related to the STs most commonly associated with conjunctivitis and does not encode the genes enriched in ECC that were searched, highlighting the point that it is not the simple lack of capsule that predisposes these strains to cause conjunctivitis. The four most common STs (ST4414, ST802, ST315 and ST4209) in nasopharyngeal carriage are all encapsulated (a cumulative 19.98% of 3,084 isolates), and lack all ECC-associated genes (except for a phage (cluster 1) shared only in ST4414) and were not found among our collection of 271 conjunctivitis isolates. Similar findings were seen by Croucher et al. [19] , with 1.14% of nasopharyngeal isolates being ST448 (21st most common ST), in this case representing the most common unencapsulated ST recovered in their study. Taken together, these findings highlight that prevalence in the nasopharynges does not directly correlate with conjunctival infection, in further support of the hypothesis that genes unique to ECC genomes are critical for conjunctival infection. It is unlikely that the unencapsulated cluster containing ECC members arose because of vaccine use, as has been speculated [8] , based on the extent of divergence between ECC lineages investigated herein and non-ocular lineages (an average 27,754 ±1,831 SNPs). On the basis of a recent determination of S. pneumoniae mutation rate [58] (and assuming that this measure is true for ECC members as well), the bifurcation between ECC and the main branch of the species took place ~8,400 years ago (8,385±553 years). That the rate of divergence measured for other S. pneumoniae also applies to ECC rates of change stems from a comparison of the distance between strains isolated from geographically and temporally related outbreaks in Maine and New Hampshire. With epidemiologic centers about 7 months apart, strains from the New Hampshire outbreak (ECC_1854 and ECC_1910) differ from those from the Maine outbreak (ECC_0072 and ECC_0083) 4.67±2.1 SNPs, a mutation rate of 1.43 × 10 −6 substitutions per site per year, in agreement with previous calculations 1.57 × 10 −6 substitutions per site per year [58] . This dating is similar to estimates of clade divergence in E. faecium [59] and S. aureus [60] both of which were attributed to increasing urbanization. This suggests that, in contrast to the ancestral line, there is an especially important role for person-to-person transmission in the propagation of either this lineage or the branch associated with respiratory infection. In summary, we found that five STs commonly associated with conjunctivitis (which accounted for 90% of S. pneumoniae conjunctivitis cases studied) belong to a distinct cluster of unencapsulated strains within the S. pneumoniae species. These strains are typified by substantially different features including elements exclusive to strains associated with conjunctivitis (CbpAC1, CbpAC2, NanO1 and NanO2) that may contribute to their ocular tropism. Additional features were shared with only closely related unencapsulated varieties (for example, ZmpC and SspBC2) or sporadically among distantly related unencapsulated strains (for example, SspBC1). Currently, 90% of the S. pneumoniae strains associated with conjunctivitis are not covered by existing vaccines. Furthermore, because of the extensive variation observed, vaccines under development that target conventional S. pneumoniae virulence traits (for example, CbpA) may or may not provide coverage for preventing conjunctivitis. This knowledge of conserved and variant features occurring in the ECC members will be critical for future vaccine-design strategies. Bacterial strains A large and comprehensive collection of 280 S. pneumoniae conjunctivitis strains were assembled from across the United States of America, including 271 isolates obtained from 72 different zip codes, as well as one isolate from New Delhi, India as part of a national, multicentre, passive surveillance study of bacterial conjunctivitis [5] , [6] , [7] . In addition, included were two conjunctivitis isolates (six in total) from each large outbreak occurring at Dartmouth College [10] , [12] , an elementary school in Maine [13] , [17] , and a suburb of Minnesota [9] , as well as three other conjunctivitis isolates of unknown origin were obtained from the CDC Streptococcus Laboratory ( Supplementary Data 1 ). Strains were cultured on 5% sheep blood agar plates (BD Biosciences, San Jose, CA) or in Todd Hewitt broth supplemented with 5% yeast extract, and incubated at 37 °C in 5% CO 2 . Bacterial isolates were confirmed as S. pneumoniae based on their haemolysis phenotype on blood agar plates, bile solubility and susceptibility to optochin when grown in a 5% CO 2 atmosphere [8] . Ocular isolate characterization by MLST and capsule typing Multilocus sequence typing and capsule typing were performed on the 271 strains collected from the large US multicentre trial [5] , [6] , [7] ( Fig. 1b ). Briefly, sequence types were determined based on sequences for aroE , gdh , gki , recP , spi , xpt and ddl genes [61] . The presence of capsule was determined with both OMNI serum, as well as the capsule-type-specific Pneumotest-Latex serum, both obtained from the Statens Serum Institut (MiraVista Diagnostics, Indianapolis, IN). Initial capsule typing resulting for 50 selected isolates were confirmed by the Statens Serum Institut in Denmark. A preliminary report of the distribution of MLST types has been presented previously [62] . Genome sequencing Strains isolated from three well-documented major US outbreaks in Maine, New Hampshire and Minnesota, as well as strains that were representative of the MLST sequence types most prevalent among the 271 strains collected from the multicentre US study, were selected for genome sequencing ( Supplementary Data 1 ). Briefly, total DNA was purified from a 5-ml overnight culture using the DNeasy DNA extraction kit (Qiagen, Valencia, CA). Library preparation for Illumina sequencing by Illumina was carried out using the Nextera DNA Sample Preparation kit (Illumina, San Diego, CA), according to the manufacturer’s specifications. DNA quality was verified on a Bio-Tek Synergy 2 microplate reader (Winooski, VT) before quantification using a Qubit fluorometer and dsDNA High-Sensitivity assay kit (Invitrogen, Carlsbad, CA). A transposome was used to simultaneously fragment and append adapter sequences to 50 ng of DNA per sample, followed by addition of dual-index sequences in a limited-cycle PCR step. Quality and quantity of each sample library was measured on an Agilent Technologies 2100 Bioanalyzer (Santa Clara, CA), with a target fragment size of ~300 bp. The genomes of strains ECC_0072, ECC_0083, ECC_1854, ECC_1910, SC_0381 and SC_0391 were sequenced at the St Jude Children’s Hospital Hartwell Center for Bioinformatics and Biotechnology, Memphis, TN on an Illumina GAXII sequencer, according to the manufacturer’s specifications. For all other genomes, libraries were normalized to 2 nM, multiplexed and subjected to either 150, 200 or 250 bp paired end sequencing on an Illumina MiSeq Personal Sequencer at the Mass Eye and Ear Infirmary Ocular Genomics Institute (Boston, MA), according to the manufacturer’s specifications. Genome assemblies and annotation Sequence reads were assembled de novo utilizing CLC Genomics Workbench v4.9 (CLC Bio, Cambridge, MA; Supplementary Data 3 ). On average, 3.7 million high-quality paired-end reads were collected for each strain, representing >240-fold coverage of the ~2.1-Mb genomes. Sequence reads below a quality score of 25 at any position were excluded from further analyses. All genomes compared in this study ( Supplementary Data 2 ) were annotated using the Rapid Annotation using Subsystem Technology (RAST) server [63] , and Glimmer v.3 (ref. 64 ), with comparison to family profiles in the FIGfam (protein families generated by the Fellowship for Interpretation of Genomes) release 63 database. Wherever possible, manual search of the PFAM [65] database was used to assign functions to genes annotated as hypothetical. Orthogroups and gene families Orthogroups were calculated across all of the genomes in our data set using OrthoMC [66] , with a BLAST e -value of 10 −5 and an inflation index of 2.5. Orthogroups contain orthologues, which are vertically inherited genes that likely have the same function, and also possibly paralogues, which are duplicated genes that may have different functions. Phylogenic and ANI analyses SNP-based phylogeny based on MLST allele sequence and single-copy core alignment was generated using PhyML and statistics were calculated for 1,000 bootstrap replicates [67] . To generate a MLST-based tree, DNA sequences for the seven MLST loci were concatenated and aligned for each of the 31 sequence types represented in the conjunctivitis isolates ( Fig. 2 ) and the 26 non-ocular reference genomes ( Supplementary Data 2 ). A phylogenetic tree of all genomes in our data set, including the 21 genomes newly sequenced as well as 26 reference genomes ( Supplementary Data 2 ), was generated using all 1,160 single-copy core orthogroups, including S. mitis strain B6 as an outgroup. The BRAT NextGen analysis was conducted on the 1,160 single-copy core orthogroup alignment of the 47 S. pneumoniae genomes to identify the filtered-out recombinogenic regions [19] , [68] . Percent ANI was calculated by dividing the number of identical nucleotide residues in shared genes by the total number of nucleotides in shared genes [21] . Shared gene content between strains in pairwise genome comparisons was generated by searching the CDS predictions from one genome annotation against the annotations of the second genome and conserved genes were identified by BLAST matching >60% overall sequence identity [21] . Identification of antibiotic resistance genes The Resfinder database was used to identify candidate antibiotic resistance genes as described previously [69] . For a subset of the isolates, susceptibility was tested in microtitre plates and minimum inhibitory concentrations were determined by broth microdilution according to the procedure recommended by the Clinical and Laboratory Standards Institute. Western blot Logarithmically growing cells (optical density (OD) 600 =0.5) were pelleted with centrifugation and subjected to lysis in 0.1% Triton X-100. To ensure equal loading, protein concentration was determined for each lysate via absorbance at 280 nm and loaded accordingly. Duplicate gels stained with Coomasie were used to confirm equivalent loading. Lysates were run on 10% NuPAGE Bis-Tris gels (Invitrogen). Proteins were subsequently transferred to polyvinylidene fluoride membranes using western blot analysis. CbpA was detected using three monoclonal antibodies (1:5,000) in PBS-T/5% non-fat dry milk. The three monoclonal antibodies (14A3, 3G12 and 3H11) recognize the highly conserved loop regions in the R2 domain of CbpA and were generated as previously described [34] . Pneumolysin was detected using rabbit polyclonal serum generated against recombinant pneumolysin. Secondary horseradish peroxidase (HRP)-conjugated antibodies (Bio-Rad, Hercules, CA) were used at 1:5,000 in PBS-T/5% non-fat dry milk. Images of the complete western blots are provided in Supplementary Fig. 8 . Aggregation assays with gp-340 Bacterial isolates (ST448, ECC_3540 and ST199, SC_3526) were cultured overnight in Todd Hewitt broth, pelleted after centrifugation (5,000 × g for 10 min), washed twice in PBS and resuspended to an OD at OD 600 =0.6 in PBS. Bacterial suspensions (300 μl) were incubated in 5 ml culture tubes in an orbital shaker at 300 r.p.m. for 1 h at 37 °C with 0, 0.5 and 1.0 μg ml −1 of purified gp-340 (DMBT-1 recombinant human protein, Life Technologies). Tubes were then rested for 1 h at 37 °C to allow bacterial aggregates to settle. Gram staining was performed for each reaction to demonstrate bacterial aggregation and representative images were acquired using an Olympus BX60 microscope. Characterization of ECC genes in nasopharyngeal genomes Additional genomes of nasopharyngeal isolates were analysed for genes found in our original data set to be specific to ECC genomes including: (a) 29 additional representatives of strains known to be associated with ECC (23 ST448, 4 SLV448, 1 ST344 and 1 ST2315), (b) 19 representatives of STs closely related to those associated with ECC, (c) 44 unencapsulated STs not closely related to ECC members were analysed ( Supplementary Data 7 ), (d) 4 encapsulated STs that were most prevalent in Chewapreecha et al. [41] This included all unencapsulated nasopharyngeal genomes in Croucher et al. [19] (16 genomes) and eight draft genomes of nasopharyngeal isolates currently available from either the NCBI GenBank or European Nucleotide Archive, including five genomes newly deposited to NCBI GenBank [70] . When available, we maximized the diversity of this set by downloading several representatives, spanning various dates of isolation, or when additional information on strain diversity was available (for example, Bayesian Analysis of Population Structure [41] ). Genomes were downloaded from the European Nucleotide Archive read archive and assembled using CLC Genomics Workbench as described above. All together, an additional 96 genomes of nasopharyngeal origin were selected to serve as a local BLAST database, which was used to search (>80% query coverage, >80% nucleotide identity) for the presence of genes identified as specific to the ECC genes in our original data set ( Supplementary Data 7 ). Accession codes : Draft genome sequences have been deposited in the DDBJ/EMBL/GenBank databases under BioProject PRJNA229402 . See Supplementary Data 2 for individual accession codes for the draft genome sequences. How to cite this article: Valentino, M. D. et al. Unencapsulated Streptococcus pneumoniae from conjunctivitis encode variant traits and belong to a distinct phylogenetic cluster. Nat. Commun. 5:5411 doi: 10.1038/ncomms6411 (2014).